MRTF-A controls vessel growth and maturation by increasing the expression of CCN1 and CCN2 Gradual occlusion of coronary arteries may result in reversible loss of cardiomyocyte function (hibernating myocardium), which is amenable to therapeutic neovascularization. The role of myocardin-related transcription factors (MRTFs) co-activating serum response factor (SRF) in this process is largely unknown. Here we show that forced MRTF-A expression induces CCN1 and CCN2 to promote capillary proliferation and pericyte recruitment, respectively. We demonstrate that, upon G-actin binding, thymosin ß4 (Tß4), induces MRTF translocation to the nucleus, SRF-activation and CCN1/2 transcription. In a murine ischaemic hindlimb model, MRTF-A or Tß4 promotes neovascularization, whereas loss of MRTF-A/B or CCN1-function abrogates the Tß4 effect. We further show that, in ischaemic rabbit hindlimbs, MRTF-A as well as Tß4 induce functional neovascularization, and that this process is inhibited by angiopoietin-2, which antagonizes pericyte recruitment. Moreover, MRTF-A improves contractile function of chronic hibernating myocardium of pigs to a level comparable to that of transgenic pigs overexpressing Tß4 (Tß4tg). We conclude that MRTF-A promotes microvessel growth (via CCN1) and maturation (via CCN2), thereby enabling functional improvement of ischaemic muscle tissue. Chronic ischaemic disease of the heart or peripheral muscle is currently treated by surgical or interventional efforts to revascularize the stenosed or occluded vascular networks. However, within a growing patient population, conventional therapeutic strategies are exhausted and clinical benefit is expected from adjuvant neovascularization therapies (angiogenesis/arteriogenesis). Previous preclinical [1] and clinical studies [2] failed to demonstrate a gain of perfusion when enforcing angiogenesis (capillary growth) in the absence of microvessel maturation—that is, recruitment of pericytes and smooth muscle cells [3] , [4] . Moreover, arteriogenesis (collateral growth), an essential element of flow improvement, did not prolong walking time in patients with critical limb ischaemia, when auxiliary granulocyte–macrophage colony-stimulating factor treatment was employed without induction of microvessel growth and stabilization [5] . In contrast, adaptive collateralization [6] occured when a pro-angiogenic factor such as vascular endothelial growth factor A (VEGF-A) was combined with the maturation factors platelet-derived growth factor-B [1] or Angiopoietin-1 (ref. 7 ). On the other hand, inhibition of NFκB signalling, impairing VEGF-A and platelet-derived growth factor-B expression, led to a hyperbranched and immature collateral network [8] . Thus, an increase in stable and regulated microvessels is required to induce functional neovascularization. Myocardin-related transcription factors (MRTFs) have been shown to activate serum response factor (SRF) [9] , [10] , [11] upon dissociation from G-actin [12] , providing muscle growth and regeneration [13] , [14] . SRF is co-activated by myocardin [15] or MRTFs A and B [16] . These SRF coactivators are interacting with G-actin and translocate to the nucleus [17] , when G-actin levels decrease, for example, due to sequestration by the G-actin-binding peptide thymosin ß4 (Tß4) [18] , [19] , [20] . Since Tß4 is a potent pro-angiogenic factor [21] , an involvement of the Tß4-MRTF-SRF axis in vascular growth would require transcriptional activation beyond well-known myogenic proteins [13] , [14] . However, MRTF coactivaton of SRF induces pro-angiogenic factors such as CCN1 (Cyr61) [22] and maturation factors such as connective tissue growth factor (CTGF) [23] , [24] . Moreover, SRF controls tip cell behaviour in angiogenesis [25] , [26] , indicating a role of MRTF-SRF in vascular growth and maintenance. In the current study, we sought to investigate the capability of MRTF-A and its upstream activator, Tß4, to induce functional vascular regeneration after prolonged ischaemia. We found that both Tß4 as well as MRTF-A increase the SRF-dependent genes CCN1 and CCN2 , and induce capillary growth and maturation in vivo . Of note, the microvascular alterations were followed by adaptive collateralization in rabbit hindlimb ischaemia and porcine chronic hibernating myocardium. In the latter model we could demonstrate that both, perfusion and function of the ischaemic myocardium, improve upon Tß4 or MRTF-A overexpression. T ß 4 and MRTF-A induce CCN1 and CCN2 in vitro We found ( Fig. 1a–d ) that MRFT-A induced hallmarks of angiogenesis—that is, migration and tube formation of cultured human microvascular endothelial cells—to a similar extent as Tß4. The pro-angiogenic effect of MRTF-A was dependent on the G-acting-binding motif of Tß4, as mutating this domain and annihilating G-acting binding abolished the Tß4 effect on vessel growth, as did a short-hairpin RNA (shRNA) interfering simultaneously with MRTF-A and B transcription (MRTF-shRNA) [27] . Consistently, Tß4 enhanced nuclear MRTF-A translocation ( Fig. 1e , Supplementary Fig. 1a,b ), as well as transcription of an MRTF/SRF-dependent reporter gene containing three SRF-binding sites of the c-fos promoter (p3DA.Luc, Fig. 1f ) [28] . Both, MRTF-A and Tß4, induced expression of genes involved in microvessel growth, most notably CCN1 , mediating angiogenesis [29] and CCN2 , relevant for 10T1/2 pericyte-like cell attraction [24] ( Supplementary Fig. 1c–g ). Of note, Tß4 transfection did not affect MRTF-A content ( Supplementary Fig. 1h ), unlike MRTF-A transfection. In line with CCN1/2 being downstream of MRTFs and relevant for vessel formation, interference with CCN1-shRNA prevented Tß4-induced tube formation ( Fig. 1g ), whereas CCN2-shRNA interrupted attachment of a murine pericyte-like cell line (C3H/10T1/2) to endothelial tubes in vitro ( Fig. 1h–i ). 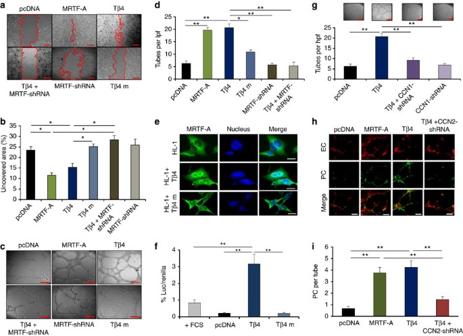Figure 1: MRTF activation and nuclear translocation induced angiogenesis via CCN1 and CCN2 activation. (a,b) MRTF-A transfection enhanced endothelial cell migration in a wound-scratch assayin vitro(red area=uncovered area, scale bar: 200 μm), and (c,d) tube formation of human microvascular endothelial cells (HMECs)in vitro(lpf=low-power field). Overexpression of Tß4, a G-actin sequestering peptide activating MRTFs, displayed a similar effect unless an MRTF-shRNA was co-applied or a Tß4 mutant (Tß4 m), which lacked the G-actin-binding motif KLKKTET, were used (scale bar: 200 μm). (e) Tß4 transfection of myocytic HL-1 cells enabled nuclear (blue fluorescence) translocation of MRTF-A (green fluorescence), an effect absent when the Tß4 m construct was used lacking the G-actin-binding site (scale bar: 20 μm). (f) Tß4 transfection of HL-1 cells induced an MRTF-SRF-sensitive luciferase reporter (containing three copies of the c-fos SRF-binding site=p3DA.Luc, cf.44), unlike Tß4 mutant transfection. (g) Tß4-induced tube formation was abolished in case of shRNA-co-transfection of the MRTF/SRF target geneCCN1 (Cyr61, scale bar: 200 μm) (h,i). Tube maturation, assessed as pericyte recruitment (PC, green fluorescence) to endothelial rings (EC rings, red fluorescence, scale bar: 200 μm) was induced by MRTF-A and Tß4. Co-transfection of shRNA versus the MRTF-target gene CCN2 (CTGF) abolished the Tß4 effect. (All error bars: mean±s.e.m.,n=5, *P<0.05, **P<0.001, using analysis of variance (ANOVA) with the Student–Newman–Keul’s procedure) Figure 1: MRTF activation and nuclear translocation induced angiogenesis via CCN1 and CCN2 activation. ( a , b ) MRTF-A transfection enhanced endothelial cell migration in a wound-scratch assay in vitro (red area=uncovered area, scale bar: 200 μm), and ( c , d ) tube formation of human microvascular endothelial cells (HMECs) in vitro (lpf=low-power field). Overexpression of Tß4, a G-actin sequestering peptide activating MRTFs, displayed a similar effect unless an MRTF-shRNA was co-applied or a Tß4 mutant (Tß4 m), which lacked the G-actin-binding motif KLKKTET, were used (scale bar: 200 μm). ( e ) Tß4 transfection of myocytic HL-1 cells enabled nuclear (blue fluorescence) translocation of MRTF-A (green fluorescence), an effect absent when the Tß4 m construct was used lacking the G-actin-binding site (scale bar: 20 μm). ( f ) Tß4 transfection of HL-1 cells induced an MRTF-SRF-sensitive luciferase reporter (containing three copies of the c-fos SRF-binding site=p3DA.Luc, cf. [44] ), unlike Tß4 mutant transfection. ( g ) Tß4-induced tube formation was abolished in case of shRNA-co-transfection of the MRTF/SRF target geneCCN1 (Cyr61, scale bar: 200 μm) ( h , i ). Tube maturation, assessed as pericyte recruitment (PC, green fluorescence) to endothelial rings (EC rings, red fluorescence, scale bar: 200 μm) was induced by MRTF-A and Tß4. Co-transfection of shRNA versus the MRTF-target gene CCN2 (CTGF) abolished the Tß4 effect. (All error bars: mean±s.e.m., n =5, * P <0.05, ** P <0.001, using analysis of variance (ANOVA) with the Student–Newman–Keul’s procedure) Full size image Role of MRTFs in Thymosin ß4-induced neovascularization To further demonstrate the relevance of MRTF signalling in vivo , we used a murine hindlimb ischaemia model. Intramuscular (i.m.) injection of recombinant adeno-associated virus (AAV) vectors (rAAVs, Supplementary Fig. 2a–c ) raised tissue concentration of target proteins in the treated limb ( Fig. 2a ) and transcript levels of the downstream mediators CCN1 and CCN2 ( Fig. 2b , Supplementary Fig. 2d–f ). Consistently, rAAV.MRTF-A induced capillary growth ( Fig. 2c,d ) and increased perfusion at d7 ( Fig. 2e,f ). As an upstream activator, Tß4 had a similar effect on vessel growth and function ( Fig. 2c–f ), unless the G-actin-binding motif was lacking (Tß4 m) or an rAAV.MRTF-shRNA was co-applied. To further assess the relevance of MRTFs in Tß4-induced vessel growth, rAAV.Cre was applied to Mrtf-a −/− Mrtfb flox/flox hindlimbs in order to cause MRTF-A and -B double deficiency. In Cre-induced MRTF-A/B knockouts, Tß4 was unable to stimulate capillary growth ( Fig. 2g ), pericyte recruitment ( Supplementary Fig. 2g,h ) and improve perfusion ( Fig. 2h , Supplementary Fig. 2i ) at d7 after ischaemia induction. Similarly, when rAAV.Cre was applied to CCN-1 flox/flox mice, hindlimbs did not display Tß4-mediated gains of either capillaries ( Fig. 2i,j ) or perfusion at d7 ( Fig. 2k,l ). Thus, MRTF-A transduction or MRTF activation via Tß4-mediated G-actin sequestration stimulate transcription of CCN1 to mediate functional vascular regeneration. 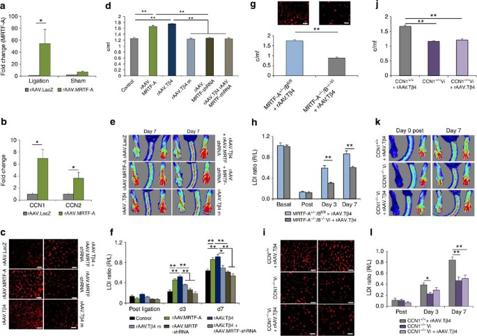Figure 2: Importance of MRTF signalling for neovascularizationin vivo. (a) qRT–PCR analysis revealed an increase in MRTF-A in the rAAV.MRTF-A-transduced ischaemic hindlimb. (b) rAAV.MRTF-A induced MRTF/SRF target genes CCN1 and CCN2in vivo. (c,d) rAAV.MRTF-A transduction increased capillary/muscle fibre ratio (c/mf), similar as the MRTF-activator Tß4. rAAV.Tß4 m, a mutant lacking the G-actin-binding domain, or co-application of Tß4 and rAAV.MRTF-shRNA had no effect (PECAM-1 staining, scale bar: 100 μm). (e,f) Functionally, rAAV.MRTF-A and -Tß4, but not rAAV.Tß4 m or rAAV.Tß4+MRTF-shRNA, transduction improved hindlimb perfusion at d3 and d7 (e). (g) After rAAV.Cre vector-induced MRTFB deletion in MRTF-A-deficient mice (Mrtf-a−/−/bflox/flox+rAAV.Cre=MRTF-A/B−/−Vi), Tß4 transduction was not capable of inducing angiogenesis, as opposed to Mrtf-a+/−/bflox/flox(=MRTF-A/B+/−)mice. (h) rAAV.Tß4-increased perfusion was abolished in MRTF-A/B−/−Vi mice. (i,j) In CCN1−/−Vi mice (=CCNflox/flox+rAAV.Cre), the increase of capillary/muscle fibre ratio was abolished (PECAM-1 staining, scale bar: 100 μm), as was the gain of hindlimb perfusion (k,l). (All error bars: mean±s.e.m.,n=5, *P<0.05, **P<0.001, using ANOVA with the Student–Newman–Keul’s procedure). Figure 2: Importance of MRTF signalling for neovascularization in vivo . ( a ) qRT–PCR analysis revealed an increase in MRTF-A in the rAAV.MRTF-A-transduced ischaemic hindlimb. ( b ) rAAV.MRTF-A induced MRTF/SRF target genes CCN1 and CCN2 in vivo . ( c , d ) rAAV.MRTF-A transduction increased capillary/muscle fibre ratio (c/mf), similar as the MRTF-activator Tß4. rAAV.Tß4 m, a mutant lacking the G-actin-binding domain, or co-application of Tß4 and rAAV.MRTF-shRNA had no effect (PECAM-1 staining, scale bar: 100 μm). ( e , f ) Functionally, rAAV.MRTF-A and -Tß4, but not rAAV.Tß4 m or rAAV.Tß4+MRTF-shRNA, transduction improved hindlimb perfusion at d3 and d7 ( e ). ( g ) After rAAV.Cre vector-induced MRTFB deletion in MRTF-A-deficient mice (Mrtf-a −/− /b flox/flox +rAAV.Cre=MRTF-A/B −/− Vi), Tß4 transduction was not capable of inducing angiogenesis, as opposed to Mrtf-a +/− /b flox/flox (=MRTF-A/B +/− )mice. ( h ) rAAV.Tß4-increased perfusion was abolished in MRTF-A/B −/− Vi mice. ( i , j ) In CCN1 −/− Vi mice (=CCN flox/flox +rAAV.Cre), the increase of capillary/muscle fibre ratio was abolished (PECAM-1 staining, scale bar: 100 μm), as was the gain of hindlimb perfusion ( k , l ). (All error bars: mean±s.e.m., n =5, * P <0.05, ** P <0.001, using ANOVA with the Student–Newman–Keul’s procedure). Full size image MRTFs induced pericyte recruitment and collateral growth The interdependence of microcirculatory growth and arteriogenesis for the mediation of flow recovery was assessed in a rabbit ischaemic hindlimb model ( Supplementary Fig. 3a ), which is compatible with topic separation of the microvessel growth area (lower limb) and the collateralization area (upper limb). Regional transduction of the ischaemic calf muscles with MRTF-A or Tß4 via rAAV ( Fig. 3a , Supplementary Fig. 3b–d ) led to functional neovascularization including CD31 + capillary sprouting, NG2 + pericyte investment ( Fig. 3b–d ) and collateral growth ( Fig. 3e,f ). Of note, MRTF activation via Tß4 transduction of the thigh region, although capable of inducing a modest collateral growth, did not increase perfusion, whereas restricting MRTF activation via Tß4 to the calf region sufficed to significantly stimulate micro- and macrovascular growth as well as perfusion ( Supplementary Fig. 3e–i ). Detachment of microvascular pericytes by forced Angiopoietin-2 expression ( Fig. 3b–d ) abrogated the Tß4- and MTRF-A-mediated collateralization and flow improvement ( Fig. 3e–g ). Moreover, blocking flow-induced vasodilation by oral application of L-NAME, an unselective nitric oxide synthase inhibitor, did not affect capillary growth and maturation ( Supplementary Fig. 3j ) but prevented collateral formation and increased perfusion ( Supplementary Fig. 3k–l ). Thus, nitric oxide appears to provide collateral growth upon microcirculatory growth and maturation. This observation is complemented by the finding that direct Tß4 injection into the area of collateral growth (upper limb) does not improve perfusion to the same extent as remote injection of rAAV.Tß4 into the lower limb, the site of microcirculatory growth ( Supplementary Fig. 3e–i ). These findings indicate that microvessel maturation and nitric oxide signalling are processes that have to occur in the sequence of MRTF-A-mediated vascular growth in order to accomplish functional vascular regeneration. 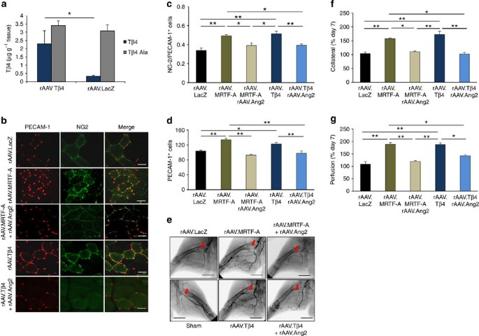Figure 3: Tß4/MRTF-A-induced microvessel maturation is essential for collateral growth and improved perfusion. (a) HPLC analysis revealed a significant increase in Tß4 protein after rAAV.Tß4 transduction of ischaemic rabbit hindlimbs, whereas rabbit-specific Tß4-Ala remained unchanged. (b–d) rAAV.MRTF-A or rAAV.Tß4 application enhanced capillary density (PECAM-1 staining) as well as pericyte investment (NG2 staining, scale bar: 50 μm), which are both abolished by co-application of Angiopoietin-2 (rAAV.Ang2). (e,f) Angiographies of ischaemic hindlimbs on day 35 revealed an increased collateral formation in rAAV.MRTF-A- and rAAV.Tß4-treated animals (red arrows indicate site of femoral artery excision, scale bar: 2 cm). Co-application of rAAV.Ang2 abolished this effect. (g) rAAV.MRTF-A and rAAV.Tß4 induced a gain of perfusion in ischaemic hindlimbs, unless rAAV.Ang2 was co-applied. (all error bars: mean±s.e.m.,n=5, *P<0.05, **P<0.001, using ANOVA with the Student–Newman–Keul’s procedure). Figure 3: T ß 4/MRTF-A-induced microvessel maturation is essential for collateral growth and improved perfusion. ( a ) HPLC analysis revealed a significant increase in Tß4 protein after rAAV.Tß4 transduction of ischaemic rabbit hindlimbs, whereas rabbit-specific Tß4-Ala remained unchanged. ( b – d ) rAAV.MRTF-A or rAAV.Tß4 application enhanced capillary density (PECAM-1 staining) as well as pericyte investment (NG2 staining, scale bar: 50 μm), which are both abolished by co-application of Angiopoietin-2 (rAAV.Ang2). ( e , f ) Angiographies of ischaemic hindlimbs on day 35 revealed an increased collateral formation in rAAV.MRTF-A- and rAAV.Tß4-treated animals (red arrows indicate site of femoral artery excision, scale bar: 2 cm). Co-application of rAAV.Ang2 abolished this effect. ( g ) rAAV.MRTF-A and rAAV.Tß4 induced a gain of perfusion in ischaemic hindlimbs, unless rAAV.Ang2 was co-applied. (all error bars: mean±s.e.m., n =5, * P <0.05, ** P <0.001, using ANOVA with the Student–Newman–Keul’s procedure). Full size image Efficacy of MRTF-A resolving hibernating myocardium Although peripheral and coronary arteries both perfuse muscle tissue, a unique feature of the heart muscle is its permanent contractile activity that requires continuous oxygen supply. A chronic decrease in oxygen supply alters the cellular composition of viable cardiomyocytes in the ischaemic area, resulting in a regional loss of contractile force called hibernating myocardium [30] , [31] . Inside cardiomyocytes, hallmarks of hibernating myocardium are reduced myofilaments [32] and mitochondria content as well as an increased glycogen content [33] . Here we studied the potential of MRTF-A to resolve dysfunction in hibernating myocardium because of percutaneous implantation of a reduction stent in pig hearts [34] inducing gradual occlusion of the Ramus Circumflexus (RCx, Supplementary Fig. 4a ). At d28 after rAAV.MRTF-A application into the ischaemic area, significantly increasing MRTF-A tissue content ( Supplementary Fig. 4b ), we found a significantly higher degree of capillary density and pericyte coverage ( Fig. 4a–c ). Collateral growth and perfusion under rapid pacing (130 min −1 ) were still impaired at d28—that is, before LacZ- and MRTF-A transduction ( Supplementary Fig. 4c–f )—but improved at d56—that is, 4 weeks after MRTF-A-, and not LacZ transduction ( Fig. 4d–f ). 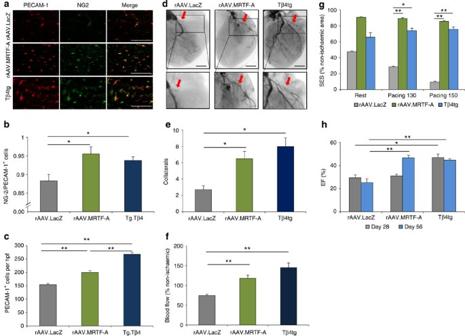Figure 4: MRTF-A improves collateral formation and perfusion in the hibernating pig myocardium. (a–c) In hibernating porcine myocardium (cf.Supplementary Fig. 4a), rAAV.MRTF-A transduction as well as ubiquitous overexpression of Tß4 (Tß4tg, cf.Supplementary Fig. 5) induced capillary sprouting (PECAM-1 staining, scale bar: 50 μm) as well as pericyte investment (NG2 staining). (d,e) Moreover, collateral growth was detected in rAAV.MRTF-A-transduced hearts, similar to Tß4tg hearts (scale bar: 2 cm). (f) Regional flow reserve, obtained at rapid atrial pacing (130 beats per minute), was found to be increased in rAAV.MRFT-A-transduced and Tß4-transgenic hearts. (g) Regional myocardial function, assessed by subendocardial segment shortening at rest and under atrial pacing (130 and 150 beats per minute), revealed an improved functional reserve by either via rAAV.MRTF-A transduction or in Tß4tg hearts. (h) Ejection fraction, a parameter of global myocardial function, improved in rAAV.MRTF-A-transduced animals on day 56 compared with day 28. In contrast, constitutively Tß4-overexpressing animals (Tß4tg) displayed no loss of function on day 28. (All error bars: mean±s.e.m.,n=5, *P<0.05, **P<0.001, using ANOVA with the Student–Newman–Keul’s procedure). Figure 4: MRTF-A improves collateral formation and perfusion in the hibernating pig myocardium. ( a – c ) In hibernating porcine myocardium (cf. Supplementary Fig. 4a ), rAAV.MRTF-A transduction as well as ubiquitous overexpression of Tß4 (Tß4tg, cf. Supplementary Fig. 5 ) induced capillary sprouting (PECAM-1 staining, scale bar: 50 μm) as well as pericyte investment (NG2 staining). ( d , e ) Moreover, collateral growth was detected in rAAV.MRTF-A-transduced hearts, similar to Tß4tg hearts (scale bar: 2 cm). ( f ) Regional flow reserve, obtained at rapid atrial pacing (130 beats per minute), was found to be increased in rAAV.MRFT-A-transduced and Tß4-transgenic hearts. ( g ) Regional myocardial function, assessed by subendocardial segment shortening at rest and under atrial pacing (130 and 150 beats per minute), revealed an improved functional reserve by either via rAAV.MRTF-A transduction or in Tß4tg hearts. ( h ) Ejection fraction, a parameter of global myocardial function, improved in rAAV.MRTF-A-transduced animals on day 56 compared with day 28. In contrast, constitutively Tß4-overexpressing animals (Tß4tg) displayed no loss of function on day 28. (All error bars: mean±s.e.m., n =5, * P <0.05, ** P <0.001, using ANOVA with the Student–Newman–Keul’s procedure). Full size image Enhanced collateral perfusion ( Supplementary Fig. 4g ) generated an improved functional reserve of the ischaemic area at rapid pacing (130 and 150 beats per minute, Fig. 4g ). Concomitantly, we found an improved ejection fraction (EF) as marker of global systolic function ( Fig. 4h , dynamic examples in Supplementary Fig. 4 and Supplementary video 1,2 ) and a decrease in the left ventricular end diastolic pressure ( Supplementary Fig. 4i ), a prognostic marker of beginning heart failure. Transgenic pigs ubiquitously and constitutively overexpressing Tß4 ( Supplementary Fig. 5 ) displayed similar capillary growth and maturation as rAAV-MRTF-A-treated animals ( Fig. 4a–c ). At d56, the blood flow reserve in the ischaemic area was increased ( Fig. 4f ), and functional reserve of either the ischaemic region ( Fig. 4g ) or the whole heart ( Fig. 4h ) was enhanced as in rAAV.MRTF-A-treated hearts. Of note, by virtue of the constitutive Tß4 overexpression already from days 0 to 28, Tß4tg animals did not experience a significant loss of perfusion nor myocardial function at rest or under rapid pacing ( Fig. 4g , Supplementary Fig. 4d–g,i ). Moreover, rAAV.Tß4-induced micro- and macrovascular growth and subsequent increases in perfusion reserve were abrogated, when an inhibitory MRTF-A-shRNA was co-applied (Fig. 5a–g ). The gain of global ( Fig. 5h , dynamic examples in Supplementary video 3,4 ) and regional myocardial function ( Fig. 5i ) was abolished when Tß4 transduction was combined with MRTF-A inhibition by a suitable shRNA. 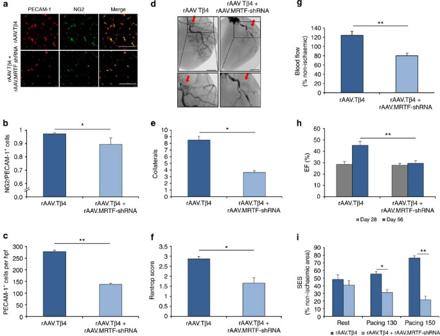Figure 5: MRTFs are required for Tß4-induced cardioprotection. (a,b) rAAV.Tß4 induced capillary growth (PECAM-1 staining) and (c) pericyte investment (NG2 staining; scale bar: 50 μm), unless co-application of rAAV.MRTF-shRNA abrogated both processes. (d,e) Collateral growth was detected in rAAV.Tß4-transduced animals but not after co-application of rAAV.MRTF-shRNA (scale bar: 2 cm). (f) Rentrop score revealed an enhanced collateralization after rAAV.Tß4 transduction, except in case of MRTF-A-shRNA co-application. (g) Regional myocardial blood flow at flow reserve (atrial pacing 130 min−1) improved in rAAV.Tß4-treated animals but not in rAAV.Tß4+MRTF-shRNA hearts. (h) Analysis of ejection fraction revealed an improvement of systolic myocardial function in rAAV.Tß4-transduced animals (d56), compared with day 28 (day of transduction). No gain of ejection fraction was found in rAAV.Tß4+MRTF-shRNA-treated hearts. (i) Regional myocardial function, assessed by subendocardial segment shortening at rest and under atrial pacing (130 and 150 bpm), reveals an increased functional reserve after rAAV.Tß4-, but not rAAV.Tß4+MRTF-shRNA transduction. (All error bars: mean±s.e.m.,n=5, *P<0.05, **P<0.001, usingt-test for comparison of two groups or ANOVA with the Student–Newman–Keul’s procedure for multiple group comparison). Figure 5: MRTFs are required for T ß 4-induced cardioprotection. ( a , b ) rAAV.Tß4 induced capillary growth (PECAM-1 staining) and ( c ) pericyte investment (NG2 staining; scale bar: 50 μm), unless co-application of rAAV.MRTF-shRNA abrogated both processes. ( d , e ) Collateral growth was detected in rAAV.Tß4-transduced animals but not after co-application of rAAV.MRTF-shRNA (scale bar: 2 cm). ( f ) Rentrop score revealed an enhanced collateralization after rAAV.Tß4 transduction, except in case of MRTF-A-shRNA co-application. ( g ) Regional myocardial blood flow at flow reserve (atrial pacing 130 min −1 ) improved in rAAV.Tß4-treated animals but not in rAAV.Tß4+MRTF-shRNA hearts. ( h ) Analysis of ejection fraction revealed an improvement of systolic myocardial function in rAAV.Tß4-transduced animals (d56), compared with day 28 (day of transduction). No gain of ejection fraction was found in rAAV.Tß4+MRTF-shRNA-treated hearts. ( i ) Regional myocardial function, assessed by subendocardial segment shortening at rest and under atrial pacing (130 and 150 bpm), reveals an increased functional reserve after rAAV.Tß4-, but not rAAV.Tß4+MRTF-shRNA transduction. (All error bars: mean±s.e.m., n =5, * P <0.05, ** P <0.001, using t -test for comparison of two groups or ANOVA with the Student–Newman–Keul’s procedure for multiple group comparison). Full size image Here using a combined genetic and physiological approach in mouse, rabbit and pig models, we show that MRTFs stimulate growth and maturation of microvessels as well as increased collateral blood flow upon arterial occlusion in hindlimb and coronary networks. Mechanistically, we demonstrate that MRTF translocation downstream of Tß4 coactivates SRF inducing CCN1/CCN2 resulting in augmented angiogenesis and vascular smooth muscle cell recruitment and formation of functional vessels that can carry collateral flow ( Fig. 6 ). 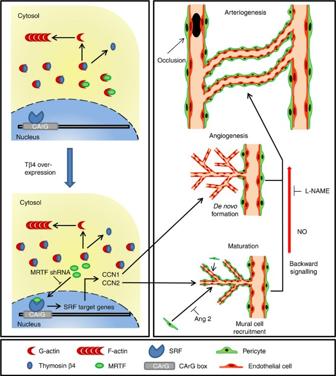Figure 6: Mechanisms of MRTF-mediated therapeutic neovascularization. MRTF-A or Tß4 transduction induces an increased amount of MRTF-A unbound to G-actin, which after translocation to the nucleus interacts with SRF, inducing, for example, CCN1 and CCN2 as target genes. CCN1 enables capillary growth (angiogenesis), whereas CCN2 enhances the pericyte investment (vessel maturation). Together, these mechanisms induce collateral growth in a nitric oxide-dependent manner leading to a therapeutic neovascularization. Figure 6: Mechanisms of MRTF-mediated therapeutic neovascularization. MRTF-A or Tß4 transduction induces an increased amount of MRTF-A unbound to G-actin, which after translocation to the nucleus interacts with SRF, inducing, for example, CCN1 and CCN2 as target genes. CCN1 enables capillary growth (angiogenesis), whereas CCN2 enhances the pericyte investment (vessel maturation). Together, these mechanisms induce collateral growth in a nitric oxide-dependent manner leading to a therapeutic neovascularization. Full size image Of note, the relevance of the Thymosinß4/MRTF-A/SRF pathway for microcirculatory growth was demonstrated, since deletion of CCN1 , a gene induced by this transcriptional pathway, abrogated the gain of vascular structures and function in vivo . Moreover, in rabbit and pig models, we extend this notion to the formation of collaterals upon microcirculatory growth, a property not universal to vascular growth factors. A key feature of MRTF-A activation is nuclear translocation upon reduction in G-actin levels, and nuclear export when G-actin abundance increases [10] , [35] . Forced expression of MRTF-A or Tß4, a peptide activating MRTF-A by G-actin binding ( Fig. 1 ), initiates an orchestrated micro- and macrocirculatory growth response in case of chronic peripheral ( Figs 2 and 3 ) and heart ( Fig. 4 ) muscle ischaemia. Consistently, chronic dysfunction of hibernating pig myocardium was resolved by either direct MRTF-A overexpression or MRTF-A activation via Tß4 ( Fig. 4 ). The notion that MRTF-A-SRF signalling provides myofilaments is of particular interest since a loss of actin cytoskeleton is a hallmark of hibernating myocardium caused by chronic coronary hypoperfusion [32] . Thus, MRTF-A is located at the crossroads of myocyte and vessel regeneration in hibernating myocardium. Tß4, the most abundant G-actin-binding peptide of the cytosol, is capable of inducing vessel growth via endothelial migration and sprouting [21] , [36] . An essential role of MRTF-A in Tß4 angiogenic signalling was established in vitro and in vivo , since MRFT-A-shRNA was capable of abrogating endothelial migration and sprouting ( Fig. 1b,d ) as well as micro- and macrovascular growth ( Fig. 2d,f ) and functional cardiac improvement ( Supplementary Fig. 6 ). Accordingly, endothelial-specific deficiency of MRTFs caused incomplete formation of the primary vascular plexus of the developing retina [26] . Moreover, SRF, the main target of MRTF-A, has recently been identified as crucial for tip cell behaviour in sprouting angiogenesis upon VEGF-A stimulation [25] . Nevertheless, VEGF-A results in growth of immature and unstable capillaries [37] , as opposed to Tß4-MRTF-A, pointing to a difference in signalling of both vessel growth factors. A particular feature of the Tß4-MRTF-A-SRF signalling axis is the balanced nature of vascular growth—that is, microvessel growth and maturation as well as adaptive collateralization. Surprisingly, angiopoietin-2 not only abrogated pericyte investment after MRTF-A- or Tß4 treatment ( Fig. 3b,c ) but also compromised adaptive collateralization ( Fig. 3e–g ). Thus, microcirculatory maturation appears to be essential for the transmission of collateral growth signals. The role of the microvascular compartment is additionally underscored by the observation that local i.m. treatment of the collateral compartment (upper limb in rabbits) does not provide an equivalent vascular regeneration to local i.m. treatment of the microvascular compartment (lower limb, Supplementary Fig. 3g–i ). An essential signal, sent from the microvascular compartment to induce adaptive collateral growth, appears to be nitric oxide, since the unselective nitric oxide synthase inhibitor L-NAME abrogated the arteriogenic effect of Tß4. Of note, L-NAME did not affect capillary sprouting nor pericyte to endothelial cell ratio in Tß4-treated hindlimbs ( Supplementary Fig. 3j–l ). These experiments indicate a hierarchical order in the balanced vascular growth process induced by the Tß4-MRTF-A-SRF axis, which originates in the microvasculature and progresses to subsequent adaptive collateralization. Collectively, our data demonstrate that activation of Tß4-MRTF augments collateral blood flow in ischaemic heart and hindlimb via induction of CCN1/CCN2. At the cellular level this response involves endothelial sprouting via CCN1 (CYR61) [29] and maturation—that is, pericyte investment—via CCN2 (CTGF) [24] resulting in a stable and functional vascular network that can carry collateral blood flow and improve conductance. Pericyte investment is crucial herein since Ang 2, by virtue of disrupting pericyte investment [38] , abolished the positive effects exerted by Tß4-MRTF signalling ( Fig. 3 ). This finding indicates the central role of vessel maturation and balanced vessel growth and paves new therapeutic avenues towards functional neovascularization. Reagents All cell culture media and chemicals were purchased from Sigma (Deisenhofen, Germany) if not indicated otherwise. Contrast agent Solutrast 370 was provided by Byk Gulden (Konstanz, Germany). CCN1-shRNA (Cyr61-shRNA, sc-39332) and CCN2-shRNA (CTGF-shRNA, sc-39329) were purchased from Santa Cruz Biotechnology, CA, USA. Adeno-associated viral vectors The recombinant rAAV.MRTF-A, rAAV.Tß4, rAAV.Tß4m, rAAV.LacZ, rAAV.Cre and rAAV.MRTF-shRNA (5′-GATCCCCGCATGGAGCTGGTGGAGAAGAATTCAAGAGATTCTTCTCCACCAGCTCCATGTTTTTGGAAA-3′) vectors were produced using triple transfection of U293 cells. One plasmid encoded the transgene under control of a CMV promoter flanked by cis -acting AAV2 internal terminal repeats, a second plasmid provided AAV2 rep and AAV9 cap in trans [39] , whereas a third plasmid (delta F6) supplemented adenoviral helper function. Cells were harvested 48 h later and vectors purified with caesium gradients [40] . Viral titres were determined using RT–PCR against the polyA tail of the vector bGH (primer sequence see Table 1 ). Trans and helper plasmids were kindly provided by James M. Wilson, University of Pennsylvania. Table 1 Primer sequences used for PCR were as follows. Full size table Cell culture Satisfection (TPP AG, Trasadingen, Schweiz) was used for the transfection of human microvascular endothelial cells (HMECs, CDC, North Carolina, USA), murine endothelial cells (bEnd.3, CRL-2299, ATCC, USA) and myocytic cell line (HL-1 cells, kindly provide by Dr W. Claycomb) according to the manufacturer’s instructions. Here 100 μl serum- and antibiotic-free DMEM medium were mixed with 3 μl Satisfection transfection agent. In vitro tube formation and coculture experiments For matrigel experiments, HMECs were transfected with pcDNA, MRTF-A, Tß4±MRTF-shRNA (5′-GATCCCCGCATGGAGCTGGTGGAGAAGAATTCAAGAGATTCTTCTCCACCAGCTCCATGTTTTTGGAAA-3′), Tß4 m (which lacked the G-actin-binding motif KLKKTET) [41] or Tß4±CCN1-shRNA. Cells (8,000 cells per well) were seeded on matrigel (BD Matrigel Basement Membrane Matrix, BD Biosciences, USA) in basal endothelial growth medium with an 5% fetal bovine serum addition and pictures were taken after 18 h. Number of rings per low-power field was quantified. In coculture experiments, HL-1 cells were transduced by a rAAV-Tß4±CCN1-shRNA, rAAV.MRTF-shRNA or rAAV-Tß4 m (1 × 10 6 AAV6 particles per cell). HL-1 and matrigel-embedded HMECs (8,000 cells per well) were physically separated by a permeable membrane. After 18 h, HL-1 cells were removed and ring formation per low-power field was quantified. Pericytic CH3/10T1/2 cell (CCL-226, ATCC, USA) attraction to murine endothelial cells (bEnd.3) was assessed after transfecting the endothelial compartment with pcDNA, MRTF-A or Tß4±CCN2-shRNA using Satisfection (Agilent, Boeblingen, Germany). Endothelial cells were stained DiD (red, Vybrand) and seeded on matrigel (12,000 cells per well). After 6 h DiO (green, Vybrand)-stained pericyte-like cells (2,000 cells per well) were added and migration towards tubes was allowed for 2 h. Then, coculture pictures were taken using confocal laser microscopy (Carl Zeiss, Jena, Germany). Migration assay HMEC cells were transfected with the indicated transgenes, as described above. A total of 60,000 cells were grown to confluence in wells carrying a strip-like insert (ibidi, Munich, Germany). After 24 h, the insert was removed. Images were taken at the time points 0 and 22 h at a 10-fold magnification (low-power field), and the uncovered area analysed (Image J 1.43u, National Institute of Health (NIH), USA) HL-1 cell staining Cardiomyocytic HL-1 cells were transduced by AAVs encoding for the indicated transgenes. Then, cells were plated on μ dishes (ibidi). After 48 h, nuclei were stained with Syto62. After fixation of the cells with PFA (2%), they were permeabilized and incubated with an MRTF-A antibody (1:200, Santa Cruz Biotechnology) and a secondary antibody (1:200, Alexa 488, Invitrogen, Karlsruhe, Germany). Pictures were taken using confocal laser microscopy (Carl Zeiss), and the mean fluorescence intensity of the area of 100 nuclei, identified via Syto62, was automatically assessed with its LSM5 image browser. High-performance liquid chromatography (HPLC) analysis The determination of Tß4 was performed via HPLC analysis [42] . Briefly, tissue samples were destructed by adding 4 M perchloric acid containing 1% Thiodiethanol to a final concentration of 0.4 M . Mixtures were homogenized, incubated at 4 °C for 30 min and centrifuged for 10 min at 20,000 g . The supernatant was analysed using reverse-phase chromatography. In rabbits, endogenous and exogenous Tß4 were distinguished by detection of the rabbit-specific Tß4-Ala. Luciferase assay For determining the MRTF-dependent luciferase activity, HMEC and HL-1 cells were transfected with p3DA.Luc, an SRF reporter gene (a construct of a synthetic promoter with three copies of the c-fos SRF-binding site and a Xenopus type 5 actin TATA box plus a transcription start site inserted into pGL3=p3DA.Luc) [43] and 930 ng of either pcDNA, Tß4 or a Tß4 mutant lacking the G-actin-binding site. Comparable transfection efficacy was assured by co-transfection of 50 ng ptkRL (Renilla luciferase reporter). Cell pellets were lysed, further purified by centrifugation for 10 min at 4 °C and 13,000 r.p.m. and utilized for assessment of firefly luciferase activity and Renilla luciferase activities, which are given as ratio firefly luciferase/renilla activity [43] . RNA modulation and detection Real-time (RT-)–PCR was performed with SYBR green dye (iQ SYBR Green supermix, Bio-Rad, Munich, Germany) and measured on an iQ-Cycler (Bio-Rad). RT–PCR was performed with primers mentioned in Table 1 . Expression levels were normalized to GAPDH and displayed as fold change to the pcDNA control situation. The comparative 2-DD C t method was carried out, calculating the delta C t values for the gene of interest and the housekeeping gene and then calculating the difference between both delta C t values [44] . Western blot analysis MRTF-A For analysis of total MRTF-A protein, cell culture and tissue samples were homogenized in 1 ml lyses buffer containing 20 mM Tris, 1 mM EDTA, 140 mM NaCl, 1% Nonidet P-40 (NP-40), 0.005 mg ml −1 leupeptin, 0.01 mg ml −1 aprotinin, 1 mM PMSF, pH 7.5. Whole protein extracts (60 μg) were resolved on 10% SDS–polyacrylamide gel electrophoresis (SDS–PAGE). After electrophoresis, the proteins were electrotransferred to a polyvinylidene difluoride membrane (Millipore, Billerica, MA, USA), blocked with 5% nonfat milk in PBS-0.1% Tween-20 buffer (PBS-T) and incubated overnight at 4 °C with primary antibodies against the MRTF-A (C-19, 1:125,Santa Cruz Biotechnology). After washing of the membrane, a secondary antibody (donkey anti-goat IgG 1:5,000, horseradish peroxidase-conjugated, Santa Cruz Biotechnology) was incubated and the membrane was developed with a chemiluminescence reagent (ECL, Detection Reagents, GE Healthcare, Buckinghamshire, UK). For analysis of the nuclear versus the cytosolic MRTF-A protein content, separation was performed with the Ne-Per nuclear and cytoplasmatic extraction reagents (Thermo Scientific, Rockford, IL, USA) according to the manufacturer’s instructions. After that western blot analysis was performed, as described above. As control protein either alpha Tubulin (6A204, 1:500, Santa Cruz Biotechnology) or for the nuclear fraction Lamin B1 (ZL-5, 1:500, Santa Cruz Biotechnology) was used. Full-length images of immunoblots are shown in Supplementary Fig. 6 . Animal experiments Animal care and all experimental procedures were performed in strict accordance to the German and NIH animal legislation guidelines and were approved by the Bavarian Animal Care and Use Committee (AZ 55.2-1-54-2531-26/09, 130/08, 140/07). All animal experiments were conducted at the Walter Brendel Centre of Experimental Medicine. Murine hindlimb ischaemia Unilateral hindlimb ischaemia of the right leg [45] was performed in male age-matched C57Bl6 mice (6–8 weeks of age, Charles River, Sulzfeld, Germany) as well as in MRTF-A +/− B fl/fl , MRTF-A −/− B fl/fl , MRTF-A +/− B −/− Vi (=MRTF-A +/− B fl/fl +3 × 10E12 rAAV.cre), MRTF-A −/− B −/− Vi (=MRTF-A −/− B fl/fl +3 × 10E12 rAAV.cre) and CCN1 fl/fl mice as well as CCN1 −/− Vi mice (=CCN1 fl/fl ±rAAV.cre), generated in the laboratory of Ralf Adams, presented unpublished). Before induction of ischaemia (day −14), 3 × 10 12 rAAV virus particles were applied intramuscularly to the right leg as indicated [46] . On day 0 the left leg underwent sham operation, whereas the femoral artery was ligated in the right leg. The post-ischaemic blood flow recovery was conducted using laser doppler flow cytometry (Moor Instruments, Devon, UK). Measurements were assessed directly before and after surgery, as well as on days 3 and 7. Results are given as right to left leg ratio including subtraction of background tissue value. RT–PCR and HPLC analyses were performed on day 5 after ischaemia induction; tissue was harvested from treated and non-treated legs. Analyses of capillary density and vessel maturation were performed on day 7 in all groups via PECAM-1 (sc1506, 1:50, Santa Cruz Biotechnology) and NG-2 (in MRTF-A +/− B fl/fl mice, 1:200, Chemicon, Nürnberg, Germany) staining in frozen tissue samples of the musculus gastrocnemius and musculus adductor. Rabbit hindlimb ischaemia In female rabbits, 2–2.5 kg body weight, on day 0 the complete femoral artery of the right leg was excised [44] and rAAV application (5 × 10 12 virus particles) was performed via i.m. injection into the right limb as indicated. On days 7 and 35, angiography was performed by injection of contrast agent (Solutrast 370, Byk Gulden) into the ischaemic limb with an automatic injector (Harvard Apparatus, Freiburg, Germany). Furthermore, fluorescent microspheres (15 μm, Molecular Probes, Eugene, OR, USA) were applied for blood flow measurements in the ischaemic and non-ischaemic tissues. For blood flow analysis, tissue samples were digested as described earlier. [47] , [1] Fluorescence analysis was performed via Tecan Saphire 2 microplate reader for the emission wavelengths 680, 638, 598, 545, 515, 468 and 424 nm, depending on the fluorescent colour used. Blood flow is given as percentage day 7, right to left leg [48] . Analyses of capillary density and vessel maturation were performed via PECAM-1 (sc1506, 1:50, Santa Cruz Biotechnology) and NG-2 (1:200, Chemicon) staining in frozen tissue samples (lower limb only) of the ischaemic and non-ischaemic limbs. Pig chronic myocardial ischaemia Three-month-old, male pigs were anaesthetised and arteria carotis communis as well as vena jugularis externa are instrumented [49] . Briefly, a PTFE membrane-covered restrictor stent was implanted in the proximal RCx, leading to a 75% reduction in blood flow. Correct localization of the stent and patency of the distal vessel was ensured by injection of contrast agent [49] . On day 28, baseline measurements were obtained for global myocardial function (left ventricular end diastolic pressure, EF) and myocardial perfusion (fluorescent microspheres, 15 μm, Moelcular Probes). After that, selective pressure-regulated retroinfusion into the great cardiac vein draining the RCx-perfused myocardium was performed for 5 × 10 12 virus particles rAVV.MRTF-A and rAAV.Tß4±rAAV.MRTF-shRNA. On day 56 measurements for global myocardial function and blood flow were repeated and regional myocardial function of the ischaemic and non-ischaemic areas were obtained (at rest and under rapid pacing, 130 and 150 bpm). A post-mortem angiography was performed for collateral score calculation and Rentrop score analysis (0=no filling, 1=side branch filling, 2=partial main vessel filling, 3=complete main vessel filling). Tissue was harvested for regional myocardial blood flow analysis and immunohistology. Global myocardial function On days 28 and 56, global myocardial function (left ventricular end diastolic pressure) was assessed with Millar pressure tip catheter (Sonometrics, Ontario, Canada). A left ventricular angiogram for global myocardial function was performed on days 28 and 56. EF was obtained with planimetry of end systolic and end diastolic angiogram pictures (Image J 1.43u, NIH). Regional myocardial function On day 56, after induction of ischaemia, sternotomy was performed and ultrasonic crystals were placed subendocardially in the non-ischaemic area (LAD control region) as well as in the ischaemic area (Cx perfused area) in a standardized manner. Subendocardial segment shortening (Sonometrics) was assessed at rest and under increased heart rates (functional reserve, pacing 130 and 150 bmp) and evaluated offline (electrocardiogram-dependent). Regional myocardial blood flow Analysis of the regional myocardial blood flow was performed on day 28 (before rAAV treatment) and day 56 (28 days after rAAV treatment) via fluorescent microspheres (Molecular Probes). The microspheres (15 μm, 5 × 10 6 particles per injection) were injected via a pigtail catheter into the left ventricle. Blood flow measurements were performed at rest and under increased heart rate (130 bpm). Fluorescence content was analysed via Tecan Saphire 2 micro plate reader and calculation of the regional myocardial blood flow was performed, either as ml g −1 tissue absolute or as the ratio to the non-ischaemic region at rest (blood flow % non-ischaemic) [1] , [50] . Histology Tissue samples of the ischaemic and non-ischaemic areas were analysed for capillary density (PECAM-1-positive cells, red) and pericyte investment (NG2-positive cells, green). Staining for capillaries was performed with a CD31 (PECAM-1)-antibody (1:200, SC1506, Santa Cruz Biotechnology) and a Rhodamin-labelled secondary antibody (1:50, SC2092, Santa Cruz Biotechnology), whereas the vessel maturation was quantified by pericyte (NG2 antibody, 1:200, AB5320 Millipore) co-staining. Pictures of the ischaemic and non-ischaemic regions were taken with high-power field magnification (40-fold) and five independent pictures per region (ischaemic and non-ischaemic) and per animal were quantified. rAAV transduction efficacy For evaluation of the rAAV transduction efficacy, the control mice, rabbit and pigs were treated with rAAV.LacZ. Cryosections of the LacZ-transduced animals were performed and stained for beta-galactosidase (blue staining). Furthermore, RT–PCR for the different transgenes was performed using the primers described in Table 1 and was analysed as described above. Tomato mice These mT (membrane-targeted tdTomato)/mG (membrane-targeted enhanced green fluorescent protein) homozygous expressing mice (Jackson Laboratory, Bar Harbor, ME, USA) carry loxP sites on both sides of the mT and mG encoding sequence. Cre expression via rAAV.cre for virus transduction efficacy deleted the mT (red fluorescence) in the cells and allowed for eGFP expression (green fluorescence) in the same cells ( Supplementary Fig. 2b ). Statistical methods The results are given as mean values±s.e.m. Statistical analysis for comparison of two groups was performed with Student’s t -test. Statistical analyses for multiple comparisons were performed using one-way analysis of variance. Whenever a significant effect was obtained ( P <0.05), we used multiple comparison tests between the groups with the Student–Newman–Keul’s procedure (IBM SPSS 19.0, IBM Chicago, IL, USA). Differences between groups were considered significant for P <0.05. How to cite this article : Hinkel, R. et al . MRTF-A controls vessel growth and maturation by increasing the expression of CCN1 and CCN2. Nat. Commun. 5:3970 doi: 10.1038/ncomms4970 (2014).